BiallelicVARSvariants cause developmental encephalopathy with microcephaly that is recapitulated invarsknockout zebrafish Aminoacyl tRNA synthetases (ARSs) link specific amino acids with their cognate transfer RNAs in a critical early step of protein translation. Mutations in ARSs have emerged as a cause of recessive, often complex neurological disease traits. Here we report an allelic series consisting of seven novel and two previously reported biallelic variants in valyl-tRNA synthetase ( VARS ) in ten patients with a developmental encephalopathy with microcephaly, often associated with early-onset epilepsy. In silico, in vitro, and yeast complementation assays demonstrate that the underlying pathomechanism of these mutations is most likely a loss of protein function. Zebrafish modeling accurately recapitulated some of the key neurological disease traits. These results provide both genetic and biological insights into neurodevelopmental disease and pave the way for further in-depth research on ARS related recessive disorders and precision therapies. Aminoacyl tRNA synthetases (ARSs) play a key role in protein translation as they catalyze the attachment of specific amino acids to their cognate transfer RNA (tRNA) molecules [1] , [2] . The nuclear encoded ARS gene loci are subdivided into 17 cytoplasmic, 17 mitochondrial, and three bi-functional ARSs [3] , [4] . The canonical aminoacylation and proofreading functions of ARSs are highly conserved across species. In addition, during evolution many ARSs acquired additional domains with unique structural characteristics that are not essential for tRNA charging but account for non-canonical functions [5] , [6] . These alternative functions are critical for cellular homeostasis and include among others: regulation of signal transduction and cell migration, angiogenesis and tumorigenesis, inflammatory responses, and control of cell death [5] . This functional diversity may in part account for the association between mutations in ARS genes and a broad range of human disorders, including neurological disorders, cancer, and auto-immune diseases [2] . Both monoallelic and biallelic pathogenic variants in ARS genes, encoding dominant and recessive disease traits, respectively, have been increasingly reported in patients with various disorders that often have predominantly neurological features. Dominant heterozygous mutations in ARS genes have been identified in patients with Charcot-Marie-Tooth disease and related peripheral neuropathies, including AARS [7] , GARS [8] , HARS [9] , [10] , MARS [11] , [12] , WARS [13] , and YARS [12] , [14] . Recessive mutations have been identified in complex disorders often involving the central nervous system such as hypomyelination with brainstem and spinal cord involvement ( DARS ) [15] , leukodystrophy ( RARS ) [16] , congenital visual impairment and progressive microcephaly ( KARS ) [17] , developmental delay with progressive microcephaly and intractable seizures ( QARS ) [18] , [19] and early onset epileptic encephalopathy with myelination defect ( AARS ) [20] . Interestingly, some ARS genes have been associated with both dominant and recessive disease traits including mutations in AARS [7] , [20] , KARS [21] , and YARS [14] , [22] . In this study, we report five newly diagnosed families with biallelic variants in valyl-tRNA synthetase ( VARS ), including seven novel VARS variants. In addition, we present an in-depth description of two families previously reported in a large study on brain malformations in mainly consanguineous families wherein VARS was reported as a candidate disease gene [23] . In vitro studies with patient-derived cell lines, including enzymatic assays, and yeast complementation assays show that recessive VARS mutations most likely lead to a loss-of-protein function, i.e. loss of function (LoF) alleles. A vars knockout (KO) zebrafish model further demonstrates that deficiency of vars results in microcephaly and epileptiform activity, replicating key characteristics of the human disease. Biallelic VARS variants cause developmental encephalopathy In total, ten patients from seven families with biallelic VARS variants were identified (Fig. 1a ) [23] . All families were included through international collaborations or via the program GeneMatcher [24] . All patients had global developmental delay (DD), which was already present in the first months of life in most patients, and prior to seizure onset or unrelated to epilepsy in five patients. All patients at a sufficient age for IQ testing had severe or profound intellectual disability (ID) and were nonverbal. Only two of the nine patients who had reached the walking age were able to walk independently, though both acquired this skill only at later age. Fig. 1 Identification of VARS variants in seven families with developmental encephalophaties and in silico predictions. a Pedigrees of the seven families diagnosed with VARS mutations. b Location of the identified VARS variants on protein level (InterPro/P26640). c Ribbon cartoon model of the Thermus thermophilus VARS-tRNA complex, highlighting the residues corresponding to those substituted in the human model. d Pair-wise comparisons between the wild-type (left) and mutant (right) residues for predicted changes in local contacts with tRNA or other amino acids. Hydrogen bonds were indicated as dotted yellow lines Full size image Eight out of ten patients had epileptic seizures, with onset during the neonatal or infantile period in seven patients (mean: 6 mo, median 4.3 mo). Seizure types included generalized or bilateral tonic-clonic seizures (seven patients), myoclonia (four patients), tonic seizures (one patient), focal seizures (two patients), and atypical absences (one patient). In patient 2, migrating focal seizures were documented on EEG. In four patients more than two anti-epileptic drug regimens failed meeting the definition of drug resistance [25] . No seizures were observed in patients 4 and 5 (family III), and repeated EEGs were normal. Both siblings were reported to have a notably happy demeanor resembling Angelman syndrome, but genetic testing for this syndrome was negative. Other clinical neurological features included (axial) hypotonia (four patients), spasticity (five patients), and an ataxic gait (two patients). Three patients were reported to have significant sleep problems. Brain imaging showed cerebral atrophy in eight patients and atrophy or partial agenesis of the corpus callosum in four patients. Furthermore, hypomyelination or delayed myelination was reported in four patients. All patients had a severe, progressive microcephaly on the background of a more general failure-to-thrive. Patients 9 and 10 (carrying the same VARS variant) had additional systemic features including post-natal anemia and hepatosplenomegaly in patient 9. Patient 10 died at the age of 3 years as a consequence of septic shock with no history of immunodeficiency. A detailed summary of the clinical findings in all patients is provided in Supplementary Data 1 . All patients were referred for genetic testing with WES or whole-genome sequencing (WGS) after standard diagnostic work-up did not reveal a cause for their neurodevelopmental disorder (details available in Supplementary Notes 1 to 6 ). Three compound heterozygous VARS variants were identified in the affected members of families I (p.Leu434Val/p.Gly822Ser), II (p.Gln400Pro/p.Arg442Gln), and III (p.Leu78Argfs*35/p.Arg942Gln). Of note, in addition to the biallelic VARS variant, patient 3 also carried a rare de novo variant of uncertain significance in the brain expressed gene UBE2O which has been reported 1 time in the Exome Aggregation Constortium (ExAC) [26] (OMIM 617649, Supplementary Note 2 ). Two homozygous missense variants identified in families IV (p.Leu885Phe) and V (p.Arg1058Gln) were previously reported in a large study on brain malformations in mainly consanguineous families [23] and in families VI (Jordan ancestry) and VII (Israel/Arabic ancestry), the same, homozygous, p.Arg404Trp variant was identified. 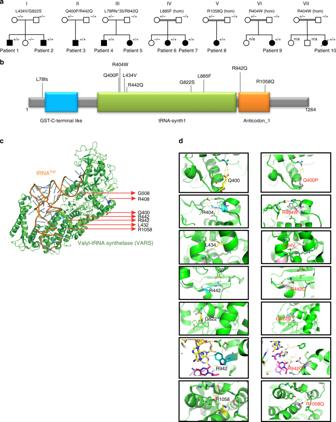Fig. 1 Identification ofVARSvariants in seven families with developmental encephalophaties and in silico predictions.aPedigrees of the seven families diagnosed withVARSmutations.bLocation of the identifiedVARSvariants on protein level (InterPro/P26640).cRibbon cartoon model of theThermus thermophilusVARS-tRNA complex, highlighting the residues corresponding to those substituted in the human model.dPair-wise comparisons between the wild-type (left) and mutant (right) residues for predicted changes in local contacts with tRNA or other amino acids. Hydrogen bonds were indicated as dotted yellow lines All VARS variants were deemed pathogenic based on their absence or presence in very low frequency in ExAC and the Genome Aggregation Database (gnomAD) [26] , impact on protein level, different prediction tools, and segregation (Supplementary Table 1 ). All identified variants were located in the catalytic or the anticodon-binding domain of the protein with the exception of the frameshift variant, which was not located in a specific domain (Fig. 1b ). In silico modeling in T. thermophilus ValRS To gain insights into the potential structural and functional consequences of the human missense variants, the sequence of the human enzyme was aligned to ValRS sequences from various taxa (Supplementary Figure 1 ), including the T. Thermophilus ValRS sequence, whose structure has been determined in complex with its cognate tRNA [27] , [28] . Of the eight VARS missense variants identified, seven could be mapped on to the corresponding residues in T. Thermophilus ValRS, allowing inferences to be drawn regarding their impact on protein structure and/or substrate interaction (Fig. 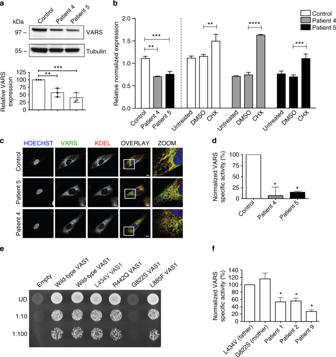Fig. 2 In vitro studies support variant pathogenicity.aWestern blot performed on patient-derived fibroblasts from patients 4 and 5 of family 3 carrying the L78Rfs*35/R942QVARSvariant showed almost 50% reduction in VARS protein. Values are mean of three separate experiments. Error bars represent SD.bRT-qPCR on the fibroblasts showed almost complete absence of the frameshift allele at mRNA level, treatment with cycloheximide caused a partial increase in expression of the frameshift allele, which was not seen with DMSO-treated control. Values are mean of three separate experiments performed in triplicate. Error bars represent SD.cImmunocytochemistry highlighted the nucleus (Hoechst), VARS and KDEL, a marker for endoplasmatic reticulum. VARS co-localizes with KDEL. There was no difference in localization between the control line and the patient fibroblasts.dVARS and TARS aminoacylation activity measured in extracts from the patient fibroblasts. The data were normalized to ATTC fibroblasts. VARS aminoacylation activity was measured in technical triplicate at three separate passages, and TARS activity was measured once in technical triplicate. Data are represented as mean-specific activity and error bars represent SEM. * indicates significant difference from control.eA haploid yeast strain deleted for endogenousVAS1was transformed with aLEU2-bearing pRS315 vector containing wild-typeVAS1, the indicated mutant form ofVAS1, or no insert (empty). Cultures for each strain (labeled along the top) were either undiluted (UD) or diluted 1:10 or 1:100 and then spotted on solid medium containing 5-FOA to determine whether theVAS1alleles complement loss of endogenousVAS1at 30 °C. Only G822S shows absent growth indicating a functional null allele.fVARS and TARS aminoacylation activity measured in extracts from patient-derived lymphoblasts of patients 1 and 2 (L434V/G822S) and their parents and patient 9 (R404W). Data were normalized to the paternal cells. VARS aminoacylation activity was measured in technical triplicate at three separate passages, and TARS activity was measured once in technical triplicate. Data are represented as mean-specific activity and error bars represent SEM. * indicates significant difference from L434V paternal lymphoid cells. Ina,b,d, andfone-way ANOVA with Tukey’s multiple comparisons test was used. Significant values are noted **p< 0.01, ***p< 0.001, and ****p< 0.0001 1c, d and Supplementary Table 2 ). Employing this analysis, the mutants fell into two different categories. The first category (6/7 variants) is composed of those substitutions that are likely to have a direct or indirect effect on protein structure, owing to a loss of a stabilizing interaction with one or more nearby residues. Substitutions falling into this category are p.Gln400Pro, p.Arg404Trp, p.Leu434Val, p.Arg442Gln, p.Gly822Ser, and p.Arg1058Gln. Prediction was weakest for p.Gln400Pro and p.Arg1058Gln as the affected residues do not make particularly strong interactions with other nearby residues. The second category (1/7) is defined by the single mutant substitution (p.Arg942Gln), which alters a direct contact to the transfer RNA substrate and, as such, could interfere with tRNA binding. The remaining variant, p.Leu885Phe, is located in an insertion in helix α13 that is missing in T. thermophilus ValRS and could not be modeled directly. Inspection of the structure of the complex suggests that this is located potentially close to the N4 of the tRNA anticodon nucleotide C38 in the bound complex and may affect one or more direct contacts to anticodon functional groups. In vitro modeling in yeast and patient-derived cell lines Fibroblast lines of the two siblings of family III (patients 4 and 5) with the compound heterozygous p.Leu78Argfs*35/p.Arg942Gln variants were available for functional testing. Both cell lines showed a statistically significant approximately twofold decrease in VARS protein compared to a control line (Fig. 2a , p < 0.001, one-way ANOVA). We hypothesized that this observation was consistent with nonsense mediated mRNA decay (NMD) of the mRNA bearing the frameshift allele and experimentally tested this hypothesis by performing RT-qPCR before and after the fibroblasts were treated with a translation inhibitor, cycloheximide (CHX) [29] . In the patient fibroblasts there was a clear absence of the frameshift allele at the cDNA level, which could be reversed by CHX treatment (Fig. 2b ). Immunofluorescence staining further demonstrated that VARS is predominantly ER-associated and that this localization was retained in patients 4 and 5 (Fig. 2c and Supplementary Figure 2 ). Extracts from these cell lines were further assessed for their ability to support aminoacylation. VARS activity from these mutated cell lines was significantly reduced (<25%) relative to control fibroblasts, whereas TARS activity was not, demonstrating that the observed reduction in enzymatic activity was VARS specific (Fig. 2d ). Fig. 2 In vitro studies support variant pathogenicity. a Western blot performed on patient-derived fibroblasts from patients 4 and 5 of family 3 carrying the L78Rfs*35/R942Q VARS variant showed almost 50% reduction in VARS protein. Values are mean of three separate experiments. Error bars represent SD. b RT-qPCR on the fibroblasts showed almost complete absence of the frameshift allele at mRNA level, treatment with cycloheximide caused a partial increase in expression of the frameshift allele, which was not seen with DMSO-treated control. Values are mean of three separate experiments performed in triplicate. Error bars represent SD. c Immunocytochemistry highlighted the nucleus (Hoechst), VARS and KDEL, a marker for endoplasmatic reticulum. VARS co-localizes with KDEL. There was no difference in localization between the control line and the patient fibroblasts. d VARS and TARS aminoacylation activity measured in extracts from the patient fibroblasts. The data were normalized to ATTC fibroblasts. VARS aminoacylation activity was measured in technical triplicate at three separate passages, and TARS activity was measured once in technical triplicate. Data are represented as mean-specific activity and error bars represent SEM. * indicates significant difference from control. e A haploid yeast strain deleted for endogenous VAS1 was transformed with a LEU2 -bearing pRS315 vector containing wild-type VAS1 , the indicated mutant form of VAS1 , or no insert (empty). Cultures for each strain (labeled along the top) were either undiluted (UD) or diluted 1:10 or 1:100 and then spotted on solid medium containing 5-FOA to determine whether the VAS1 alleles complement loss of endogenous VAS1 at 30 °C. Only G822S shows absent growth indicating a functional null allele. f VARS and TARS aminoacylation activity measured in extracts from patient-derived lymphoblasts of patients 1 and 2 (L434V/G822S) and their parents and patient 9 (R404W). Data were normalized to the paternal cells. VARS aminoacylation activity was measured in technical triplicate at three separate passages, and TARS activity was measured once in technical triplicate. Data are represented as mean-specific activity and error bars represent SEM. * indicates significant difference from L434V paternal lymphoid cells. In a , b , d , and f one-way ANOVA with Tukey’s multiple comparisons test was used. Significant values are noted ** p < 0.01, *** p < 0.001, and **** p < 0.0001 Full size image To further assess the functional effects of pathogenicity of the identified VARS missense variants, yeast complementation assays were performed by modeling VARS variants in the S. cerevisiae ortholog, VAS1 . Complementation assays were performed for all variants that were conserved between human and yeast (p.Leu434Val, p.Arg442Gln, p.Gly822Ser, and p.Leu885Phe) on a haploid yeast strain with the endogenous VAS1 gene deleted. Viability of this strain was maintained via a URA3 -bearing vector (pRS316) with a wild-type copy of VAS1 . Wild-type VAS1 on pRS315 supported yeast growth while the empty pRS315 vector did not (Fig. 2e ) consistent with our experimental vector harboring a functional VAS1 allele and with VAS1 being an essential gene. The assays further showed that p.Leu434Val, p.Arg442Gln, and p.Leu885Phe VAS1 alleles sustained yeast growth to a level comparable to wild-type VAS1 (Fig. 2e ). In contrast, p.Gly822Ser did not support yeast cell growth at all (Fig. 2e ) consistent with p.Gly822Ser VARS being a functionally null allele. These mutants were further tested for their ability to support VARS enzymatic activity. Patient-derived lymphoblast lines were available for patients 1 and 2 carrying the p.Leu434Val/p.Gly822Ser variants, their heterozygous parents, and patient 9, who was homozygous for the p.Arg404Trp variant. As shown in Fig. 2f , VARS aminoacylation was decreased on the order of 50% in patients 1 and 2 relative to that of their parents ( p < 0.05, one-way ANOVA), whereas TARS aminoacylation was >100% of the parental values. The p.Arg404Trp homozygote (patient 9) variant showed an even greater loss of VARS activity, on order of 25% relative to the heterogeneous parental samples from family I. Development of a vars knockout zebrafish model The zebrafish genome encodes a single VARS orthologue (67% identity and 77% similarity at the amino acid level to human) with a highly conserved catalytic domain (80% identity and 89% similarity). In order to deduce the potential role of vars during development, its expression patterns were examined during early development (Fig. 3a ). vars mRNA was found to be ubiquitously expressed at 18-somite stage at 18 hours post fertilization (hpf), with more distinctive expression in the brain region and in the prospective eye as well as in the hematopoietic intermediate cell mass and somites, which was maintained till 24 hpf. From 36 hpf the expression of vars became restricted to the developing brain, and after 48 hpf it was also observed in other developing organs, including branchial arches, liver, pancreas, and intestine (Fig. 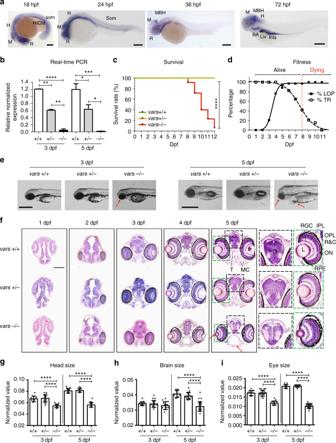Fig. 3 vars−/−larvae display severe developmental phenotype with early lethality.aSpatiotemporal expression patterns ofvarsby whole-mount RNA in situ hybridization at 18, 24, 36, and 72 hpf. BA Branchial Arches; H Hindbrain; HICM Hematopoietic Intermediate Cell Mass; Ints Intestine; Liv Liver; MBH Midbrain-Hindbrain boundary; M Midbrain; R Retina. Scale bars = 200 μmbRT-qPCR data demonstrating the expression of totalvarsinvars+/+,vars+/−, andvars−/−larvae at 3 and 5 dpf. Values are mean of three separate experiments performed in triplicate.cKaplan–Meier survival curve ofvars+/+ (n= 37),vars+/− (n= 82), andvars−/−(n= 34) larvae.dGraph illustrating changes in loss-of-posture and touch response ofvars−/−larvae throughout the life span. Only the surviving larvae were included.eRepresentative lateral and dorsal bright-field images of 3 and 5 dpfvars+/+,vars+/−, andvars−/−larvae (scale bar, 500 μm). Pericardial edema, small eye, and periocular swelling around the eye were marked with arrows.fH&E histological staining of paraffin-embedded coronary sections from the forebrain of 1–5 dpfvars+/+,vars+/−, andvars−/−larvae (scale bar, 100 μm). Magnification of the disruption in the organization of the brain and the eye for 5 dpfvars+/+,vars+/−, andvars−/−was marked with black and green stripped line, respectively. Red arrows point out some structural abnormalities. D diencephalon; IPL inner plexiform layer; L lens; MC mandibular cartilage; ON optic nerve; OPL outer plexiform layer; R&C rods and cones; RGC retinal ganglion cell; T trabecula.g–iComparison of the individual measurements for head sizeg, brain sizeh, and eye sizeiforvars+/+,vars+/−, andvars−/−at 3 dpf (n= 9,n= 20 andn= 11, respectively) and 5 dpf (n= 9,n= 14 andn= 24, respectively). Inbandg–ione-way ANOVA with Tukey’s multiple comparisons test was used. Values are mean of three separate experiments. Inclog-rank (Mantel-Cox) test was used. Error bars represent SD. Significant values are noted as ***p< 0.001 and ****p< 0.0001 3a and Supplementary Figure 3 ). These dynamic expression patterns strongly suggest an essential role of vars in the brain development, while the expression outside CNS also suggests multiple roles of vars during organogenesis. Fig. 3 vars−/− larvae display severe developmental phenotype with early lethality. a Spatiotemporal expression patterns of vars by whole-mount RNA in situ hybridization at 18, 24, 36, and 72 hpf. BA Branchial Arches; H Hindbrain; HICM Hematopoietic Intermediate Cell Mass; Ints Intestine; Liv Liver; MBH Midbrain-Hindbrain boundary; M Midbrain; R Retina. Scale bars = 200 μm b RT-qPCR data demonstrating the expression of total vars in vars +/+, vars +/−, and vars−/− larvae at 3 and 5 dpf. Values are mean of three separate experiments performed in triplicate. c Kaplan–Meier survival curve of vars +/+ ( n = 37), vars +/− ( n = 82), and vars−/− ( n = 34) larvae. d Graph illustrating changes in loss-of-posture and touch response of vars−/− larvae throughout the life span. Only the surviving larvae were included. e Representative lateral and dorsal bright-field images of 3 and 5 dpf vars +/+, vars +/−, and vars−/− larvae (scale bar, 500 μm). Pericardial edema, small eye, and periocular swelling around the eye were marked with arrows. f H&E histological staining of paraffin-embedded coronary sections from the forebrain of 1–5 dpf vars +/+, vars +/−, and vars−/− larvae (scale bar, 100 μm). Magnification of the disruption in the organization of the brain and the eye for 5 dpf vars +/+, vars +/−, and vars−/− was marked with black and green stripped line, respectively. Red arrows point out some structural abnormalities. D diencephalon; IPL inner plexiform layer; L lens; MC mandibular cartilage; ON optic nerve; OPL outer plexiform layer; R&C rods and cones; RGC retinal ganglion cell; T trabecula. g – i Comparison of the individual measurements for head size g , brain size h , and eye size i for vars +/+, vars +/−, and vars−/− at 3 dpf ( n = 9, n = 20 and n = 11, respectively) and 5 dpf ( n = 9, n = 14 and n = 24, respectively). In b and g – i one-way ANOVA with Tukey’s multiple comparisons test was used. Values are mean of three separate experiments. In c log-rank (Mantel-Cox) test was used. Error bars represent SD. 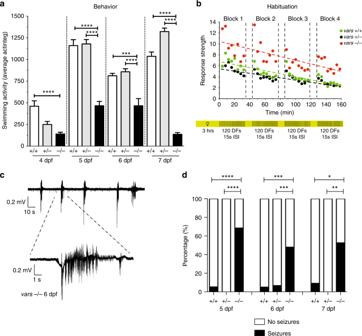Fig. 4 vars−/−larvae show cognitive deficits and spontaneous seizure like behavior.aBehavioral activity (average total movement) ofvars+/+ (n= 58),vars+/− (n= 108), andvars−/− (n= 58) larvae from 4 to 7 dpf expressed in actinteg units. Values are mean of three separate experiments.bHabituation assay performed on 6 dpfvars+/+ (n= 19),vars+/− (n= 47), andvars−/− (n= 30) larvae was composed of four blocks with 120 DFs with 15 s ISI (regions with black and yellow stripes), alternated by 10 min of light (yellow areas). The linear slopes between the actinteg responses were calculated (dotted lines) and compared between the different genotype groups (green circles—vars+/+, black circles—vars+/−, and red circles—vars−/−). DF dark flashes, ISI interstimulus intervals. Values are mean of two separate experiments.cRepresentative recording from optic tectum of 6 dpfvars−/− larva displaying polyspike discharges. Top trace represents typical pattern of epileptiform activity. Bottom trace shows magnification of the epileptiform event.dPercentage of larvae exhibiting spontaneous electrographic activity recorded from 5 dpfvars+/+ (n= 19),vars+/− (n= 31), andvars−/− (n= 35), 6 dpfvars+/+ (n= 20),vars+/− (n= 30) andvars−/−(n= 48) and 7 dpfvars+/+ (n= 12),vars+/− (n= 13) andvars−/− (n= 19) larvae. Abnormal brain activity was observed in 68.57% (24/35) 5 dpfvars−/−, 5.26% (1/19) 5 dpfvars+/+, 47.62% (23/48) 6 dpfvars−/−, 5% (1/20) 6 dpfvars+/+, 6.67% (2/30)vars+/−, 52.63% (10/19) 7 dpfvars−/−and 8.33% (1/12) 7 dpfvars+/+. Inaandbone-way ANOVA with Tukey’s multiple comparisons test was used. Ind—Fisher’s exact test was used. Significant values are noted *p< 0.05, **p< 0.01, ***p< 0.001, and ****p< 0.0001. Error bars represent SD Significant values are noted as *** p < 0.001 and **** p < 0.0001 Full size image To examine potential functional effects of VARS LoF in vivo, we generated a vars knockout model using CRISPR/Cas9 technology in zebrafish [30] , [31] (Supplementary Figure 4 ). Via RT-qPCR, we confirmed that there was an almost complete lack of total vars mRNA in vars−/− larvae at 3 and 5 days post fertilization (dpf) and approximately half of the transcript present in vars +/− larvae, proving the efficiency of the vars knockout (Fig. 3b ). Absence of vars in vars −/− larvae led to premature death between 8 and 12 dpf ( vars +/+ and vars +/− siblings remained alive), suggesting an essential role for VARS in survival (Fig. 3c ). At 7 dpf about 35.3% of vars −/− larvae showed no touch response, which was in marked contrast to the increasing touch response demonstrated by vars +/+ and vars +/− over the course of development (Fig. 3d ). Loss of posture could be observed in about 88.2% of vars −/− larvae already at 6 dpf (Fig. 3d ) and from 6 to 8 dpf ~50% of vars −/− larvae displayed abnormal motor behavior such as jerky spasmodic movements during touch response, in contrast to vars +/+ and vars+/− (data not shown). Severe morphological abnormalities were observed in vars−/− larvae from 3 dpf onwards, which were progressing over the course of time. The most prominent features were microcephaly with a partial loss of forebrain and snout, microphthalmia, and pericardial edema, as shown in bright-field images (Fig. 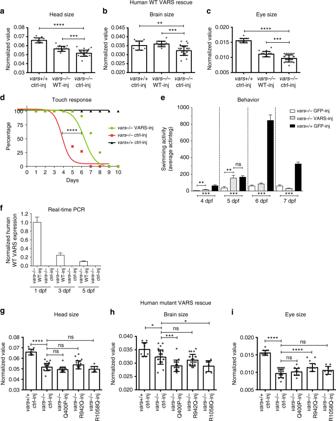Fig. 5 Wild-type humanVARSmRNA partially rescues early zebrafish phenotype, whereas mutated constructs do not.a–cComparison of the individual measurements for head sizea, brain sizeb, and eye sizecfor WT human VARS-injectedvars−/−larvae (n= 12). GFP-injectedvars+/+ larvae (n= 9) were used as a positive control, whereas GFP-injectedvars−/−larvae (n= 24) served as a negative control. Values are mean of three separate experiments.dCurves illustrating the evolution of touch response during the life span ofvars−/−larvae injected with WT humanVARS(n= 12) and GFP mRNA (n= 11) (negative control).vars−/−GFP-injected larvae were used as a positive control.eAverage total movement of WT humanVARS-injected (n= 10) and GFP-injected (n= 9)vars−/−larvae from 3 to 7 dpf.vars+/+ GFP-injected larvae (n= 14) were used as a control.fRT-qPCR data demonstrating expression levels of injected human WTVARSinvars−/−larvae at 1, 3, and 5 dpf. At 3 and 5 dpf there was 24.55% and 10.42% WTVARSmRNA left, respectively, in comparison to 1 dpf. Values are mean of three separate experiments performed in triplicate.g–iComparison of the individual measurements for head sizeg, brain sizeh, and eye sizeifor human mutated Q400P (n= 15), R942Q (n= 18) and R1058Q (n= 7) VARS-injectedvars−/−larvae. GFP-injected WT larvae (n= 9) were used as a positive control, whereas GFP-injectedvars−/−larvae (n= 24) served as a negative control. Values are mean of three separate experiments. Ina–candg–ione-way ANOVA with Tukey’s multiple comparisons test was used; ind—log-rank (Mantel-Cox) test; ine—unpairedt-test. Significant values are noted *p< 0.05, **p< 0.01, ***p< 0.001, and ****p< 0.0001. Error bars represent SD 3e and Supplementary Figure 5a ). These dysmorphologies were further investigated at the histological level on zebrafish forebrain sections from 1 to 5 dpf (Fig. 3f ). In 2 dpf vars −/− larvae, aberrant cells desquamated into the ventricular space of the forebrain and midbrain, which indicates substantial cellular changes at an early stage of development (Supplementary Data 2 ) that was not observed in the vars +/+ and vars +/− siblings. Structural abnormalities progressed over time resulting at 5 dpf in disrupted brain architecture, reduced jaw structures, delayed retinal lamination, reduced lens, and periocular swelling around the eye (corneal edema) (Fig. 3f and Supplementary Data 2 ). Measurements taken from different head areas identified significant reductions ( p < 0.0001, one-way ANOVA) in head and eye size at 3 dpf (Fig. 3g, i ), that became even more prominent at 5 dpf, where also the brain size was smaller compared to vars +/+ and vars+/− siblings (Fig. 3g–i ). To determine whether the microcephaly was due to excessive cell death in the brain, we assessed apoptosis by using antibody to active caspase-3. There were significantly more apoptotic cells detected in 3–5 dpf vars−/− brains ( p < 0.001, one-way ANOVA) than in those of their +/+ and +/− siblings (Supplementary Figure 5b ), whereas no statistically relevant difference was observed at 2 dpf. Collectively, these results suggest that loss of vars expression compromises zebrafish head and eye development and that Vars is essential for neuronal survival. Behavioral and electrophysiological studies in zebrafish Changes in behavioral activity were investigated by performing tracking experiments. vars−/− larvae showed significantly decreased swimming activity from 4 till 7 dpf ( p < 0.0001, one-way ANOVA) in comparison to vars +/+ and vars +/− (Fig. 4a ). In addition, we examined if vars−/− larvae possessed learning deficits by performing a habituation assay [32] . In the experiment, 6 dpf larvae were subjected to multiple dark flashes (DFs) alternated with light periods. Similarly to vars +/+ and vars +/−, vars −/− larvae could adapt to DFs during a training period as shown by their movement values decreasing over time (Fig. 4b ). Interestingly however, the motion of vars knockout larvae in response to DF was significantly increased ( p < 0.0001, one-way ANOVA). Fig. 4 vars−/− larvae show cognitive deficits and spontaneous seizure like behavior. a Behavioral activity (average total movement) of vars +/+ ( n = 58), vars +/− ( n = 108), and vars− /− ( n = 58) larvae from 4 to 7 dpf expressed in actinteg units. Values are mean of three separate experiments. b Habituation assay performed on 6 dpf vars +/+ ( n = 19), vars +/− ( n = 47), and vars− /− ( n = 30) larvae was composed of four blocks with 120 DFs with 15 s ISI (regions with black and yellow stripes), alternated by 10 min of light (yellow areas). The linear slopes between the actinteg responses were calculated (dotted lines) and compared between the different genotype groups (green circles— vars +/+, black circles— vars +/−, and red circles— vars− /−). DF dark flashes, ISI interstimulus intervals. Values are mean of two separate experiments. c Representative recording from optic tectum of 6 dpf vars −/− larva displaying polyspike discharges. Top trace represents typical pattern of epileptiform activity. Bottom trace shows magnification of the epileptiform event. d Percentage of larvae exhibiting spontaneous electrographic activity recorded from 5 dpf vars +/+ ( n = 19), vars +/− ( n = 31), and vars− /− ( n = 35), 6 dpf vars +/+ ( n = 20), vars +/− ( n = 30) and vars−/− ( n = 48) and 7 dpf vars +/+ ( n = 12), vars +/− ( n = 13) and vars− /− ( n = 19) larvae. Abnormal brain activity was observed in 68.57% (24/35) 5 dpf vars−/− , 5.26% (1/19) 5 dpf vars +/+, 47.62% (23/48) 6 dpf vars−/− , 5% (1/20) 6 dpf vars +/+, 6.67% (2/30) vars +/−, 52.63% (10/19) 7 dpf vars−/− and 8.33% (1/12) 7 dpf vars +/+. In a and b one-way ANOVA with Tukey’s multiple comparisons test was used. In d —Fisher’s exact test was used. Significant values are noted * p < 0.05, ** p < 0.01, *** p < 0.001, and **** p < 0.0001. Error bars represent SD Full size image To investigate whether vars knockout resulted in abnormal brain activity electrographically, we recorded local field potentials (LFPs) on larval optic tecta of 5, 6, and 7 dpf vars−/− , vars +/−, and vars +/+ zebrafish larvae. Epileptiform events were defined as multi-spike bursts with amplitudes equal to or exceeding threefold the baseline (Fig. 4c ). Recurrent spontaneous epileptiform events occurred in vars−/− at all days, being most prominent at 5 dpf where 68.57% of the larvae displayed abnormal activity, whereas no vars +/− and only 5.26% of vars +/+ showed similar events (Fig. 4d ). At 6 and 7 dpf, in 47.62 and 52.63% of vars −/− larvae, respectively, electrographic seizure activity could be detected. The morphological and behavioral phenotype of our vars−/− CRISPR model was fully recapitulated and confirmed in the vars Hi558Tg−/− zebrafish line, bearing a retroviral insertion in the first intron of vars (Supplementary Figure 6 ). Rescue experiments with human VARS mRNA To further validate the specificity of the vars knockout phenotype traits with respect to modeling neurological disease and to determine the functional consequence of selected variants identified in patients, we performed rescue experiments through mRNA injections of either wild type or mutated human VARS into vars −/− CRISPR embryos. Supplying WT VARS led to a partial or full rescue of the early phenotype in vars−/− larvae. In early development (3 dpf), a statistically significant increase for the head, brain, and eye size was observed ( p < 0.001, one-way ANOVA, Fig. 5a–c , respectively). A significantly ameliorated touch response ( p < 0.001, one-way ANOVA, Fig. 5d ), occurred in tandem with the improvement of locomotor activity being most prominent at 5 dpf (Fig. 5e ), suggesting a late response. These results were supported by the presence of exogenously supplied human WT VARS mRNA detected in vars−/− larvae at 1, 3, and 5 dpf (Fig. 5f ). Fig. 5 Wild-type human VARS mRNA partially rescues early zebrafish phenotype, whereas mutated constructs do not. a – c Comparison of the individual measurements for head size a , brain size b , and eye size c for WT human VARS-injected vars−/− larvae ( n = 12). GFP-injected vars +/+ larvae ( n = 9) were used as a positive control, whereas GFP-injected vars−/− larvae ( n = 24) served as a negative control. Values are mean of three separate experiments. d Curves illustrating the evolution of touch response during the life span of vars−/− larvae injected with WT human VARS ( n = 12) and GFP mRNA ( n = 11) (negative control). vars−/− GFP-injected larvae were used as a positive control. e Average total movement of WT human VARS- injected ( n = 10) and GFP - injected ( n = 9) vars−/− larvae from 3 to 7 dpf. vars +/+ GFP - injected larvae ( n = 14) were used as a control. f RT-qPCR data demonstrating expression levels of injected human WT VARS in vars−/− larvae at 1, 3, and 5 dpf. At 3 and 5 dpf there was 24.55% and 10.42% WT VARS mRNA left, respectively, in comparison to 1 dpf. Values are mean of three separate experiments performed in triplicate. g – i Comparison of the individual measurements for head size g , brain size h , and eye size i for human mutated Q400P ( n = 15), R942Q ( n = 18) and R1058Q ( n = 7) VARS-injected vars−/− larvae. GFP-injected WT larvae ( n = 9) were used as a positive control, whereas GFP-injected vars−/− larvae ( n = 24) served as a negative control. Values are mean of three separate experiments. In a – c and g – i one-way ANOVA with Tukey’s multiple comparisons test was used; in d —log-rank (Mantel-Cox) test; in e —unpaired t -test. Significant values are noted * p < 0.05, ** p < 0.01, *** p < 0.001, and **** p < 0.0001. Error bars represent SD Full size image In order to provide further evidence for the disease-causing nature of some of the variants, human VARS mRNA with mutant substitutions in the catalytic (p.Gln400Pro) and anticodon binding domains (p.Arg942Gln and p.Arg1058Gln) were tested for their ability to complement the vars knockout phenotype. For this experiment, we employed the early phenotype readout at 3 dpf. In contrast to the results with WT human VARS mRNA, none of the injections of human mutated VARS mRNA rescued head size or brain size of vars−/− larvae (Fig. 5g, h , respectively). Among the three variants, only the p.Arg942Gln variant provided a partial rescue of the eye size phenotype (Fig. 5i ). These observations confirmed that, despite differences in their predicted impact on VARS structure and mechanism, all three variants displayed a loss of function when tested in our vars zebrafish model. Aminoacyl-tRNA synthetases have an indispensable function in protein translation, which explains their extensive conservation throughout evolution and the fact that mutations in this class of proteins have been increasingly associated with human disease. To date, a total of 31 out of 37 ARS enzymes have been implicated in genetic diseases, which often include neurological features [2] . We studied ten patients with biallelic VARS variants and report seven new variants. Detailed clinical evaluation revealed developmental delay, early onset epilepsy, and microcephaly as key clinical characteristics. While no specific epilepsy syndrome could be associated with VARS mutations, a single patient (patient 2) had an EEG confirmed diagnosis of epilepsy of infancy with migrating focal seizures (EIMFS). Notably, this clinical diagnosis was also found in a patient with a recessive QARS mutation [18] , suggesting a potential link between this rare type of epilepsy and dysfunction of aminoacyl-tRNA synthetases. Two patients (patients 4 and 5) never manifested seizures. Interestingly, these two patients had a normal brain MRI, whereas cerebral atrophy, hypoplasia or atrophy of the corpus callosum and hypomyelination or delayed myelination were recurrent findings in the other patients. Both siblings also had severe intellectual disability to the same degree as most other VARS patients. Clinical features closely resembling the phenotype to the patients with VARS mutations described in this study have been observed for mutations in other members of the cytoplasmic ARS family, most striking in patients with biallelic mutations in QARS [18] , [19] , KARS [17] , and AARS [20] , [33] . This may indicate a joint phenotypic spectrum associated with certain aminoacyl-tRNA synthetases defects that predominantly involves developmental delay, epilepsy, and microcephaly. Interestingly, also the phenotype associated with biallelic mitochondrial VARS2 variants showed some similar features [34] . This illustrates the importance of including a broad set of genes involved in protein translation in the screening of patients with developmental (and epileptic) encephalopathies. Eight of the nine identified VARS variants were missense variants located in or near the catalytic or tRNA binding domains. The p.Leu78Argfs*35 variant, occurring in the compound heterozygous state with the p.Arg942Gln missense variant, was the only truncating VARS variant reported in our series. The frameshift allele was shown to be prone to NMD resulting in a clear decrease in expression of the mutated mRNA and protein, and decrease in VARS aminoacylation activity, consistent with a LoF allele. Immunofluorescence staining further showed that VARS is predominantly localized at the ER. This expression pattern was not altered in fibroblasts in the presence of the p.Leu78Argfs*35/p.Arg942Gln variants. To gain further insight into the pathogenic nature of the missense variants we performed predictive in silico studies of all mutations. Next, we supplemented this preliminary mutational analysis with biochemical, developmental, and neurological trait studies of selected pathogenic variant alleles in yeast, patient-derived cell lines and/or zebrafish. While a full functional characterization of each missense mutant was not performed, combined predictive and focused biochemical studies of different variants gave us sufficient information to make a statement about the pathogenic nature of most variants. Substitutions p.Gly822Ser, p.Leu434Val, p.Arg442Gln and p.Arg404Trp were each characterized by a potential destabilization of structure. While stability was not investigated directly, the results of yeast complementation analysis indicated that p.Gly822Ser clearly failed to complement, while p.Leu434Val and p.Arg442Gln were still positive for complementation. Aminoacylation assays on patient-derived cell lines further showed a clear decrease in function for p.Leu434Val, p.Gly822Ser and p.Arg404Trp. On the other hand, substitutions p.Arg942Gln and p.Leu885Phe were predicted to cause impaired recognition of substrates. The predicted tRNA binding mutant p.Arg942Gln exhibited only weak rescue of VARS function in the zebrafish knockout, and also contributed to the decreased aminoacylation seen in cell lines derived from the siblings carrying the variant. As such, this variant likely represents a hypomorphic VARS allele. The p.Leu885Phe variant was positive for yeast complementation, but was not tested for its ability to rescue the vars−/− zebrafish. Modeling analysis for the two missense variants p.Gln400Pro, and p.Arg1058Gln predicted a slightly lower likelihood of a potential protein destabilization. Nevertheless, neither p.Gln400Pro nor p.Arg1058Gln were able to rescue the zebrafish vars knockout providing experimental evidence for variant allele pathogenicity. This observation highlights the value of the zebrafish in vivo model to differentiate between pathogenic and potentially benign VARS variants with respect to the human neurological disease traits studied. Based on the above observations, we hypothesize that biallelic disease-causing VARS variants consist of a combination of a loss-of-function allele and a hypomorphic allele or alternatively a combination of two hypomorphic alleles that decrease overall VARS levels below a threshold where protein synthesis and/or other VARS-specific functions are critically threatened. Homozygosity or compound heterozygosity for null alleles would be lethal due to the essential function of VARS in all cells. Importantly, this hypothesis is supported by our observation that certain disease-associated VARS alleles retain some function. For example, p.Leu434Val VARS , when modeled in yeast, allowed cellular growth, which is expected as this mutation is opposite the functional null allele p.Gly822Ser VARS . Similarly, p.Leu885Phe VARS allowed yeast cell growth, which is expected since this allele was identified in the homozygous state. It is important to point out that our yeast assay may not be able to detect more subtle defects in enzyme function as we have shown for KARS and AARS mutations associated with recessive disease [20] , [21] . While we acknowledge the vars knockout zebrafish model is not a perfect genetic model for the human disease, we showed it accurately recapitulated many of the phenotypic features. In particular, microcephaly and epileptic activity, as seen in the patients, could also be observed in the zebrafish. Moreover, hyperactivity in vars−/− larvae observed upon light switches suggests a neuromodulatory effect, as the behavior depends on sensory input and is regulated by neuronal connectivity of the hindbrain and spinal cord and multiple neurotransmitter pathways [35] . We showed that vars was strongly and selectively expressed in the developing brain, eye and other organs during embryogenesis, as such, it is not surprising that loss of vars expression severely compromised zebrafish development. Interestingly, a qars knockout and iars knockdown zebrafish model showed some features similar to the vars model including brain malformations and extensive cell death in the brain [18] , [36] . However, the behavioral and epileptic phenotype of the qars and iars model were not further investigated and therefore cannot be compared to our model. Noteworthy, microcephaly and microphthalmia seems to be a more general phenotype associated with ARS mutations in zebrafish, since several mutant ARS lines ( kars , mars , sars , and qars ), identified in a large insertional mutagenesis screen, displayed it [37] . Our results suggest that the pathomechanism of biallelic VARS variants, and possibly of recessive ARS disease more general, is a loss-of-protein function. This contrasts with dominant mutations in ARS genes which are nearly uniformly associated with Charcot-Marie-Tooth disease, or less common peripheral neuropathies, and their functional effects likely differ (hypothesized dominant negative or gain-of-function effect) [2] . This interpretation is further supported by the fact that parents of patients with recessive VARS-associated phenotypes, who carry the mutation in a heterozygous state, are consistently reported to be phenotypically normal. Indeed, a 50% reduction in VARS activity can be tolerated without significant pathology, which is also supported by the presence of heterozygous truncating variants in public databases like ExAC and gnomAD [26] . Noteworthy, pathogenic variants in other genes that encode proteins with a prominent role in translation, can cause similar neurological disease traits to the ones associated with pathogenic variants in ARSs. For instance, CLP1 , which encodes an RNA kinase responsible for tRNA splicing required for tRNA maturation, causes microcephaly in humans, mice and zebrafish and peripheral neuropathy in humans [38] , [39] . Further studies on VARS, both in vitro and in the zebrafish model, may focus on gaining more functional insight into the underlying pathomechanism for the neurological disease traits focusing on the disrupted translational machinery and altered proteostasis or other non-canonical functions, and their effect on brain, nervous system, and global development. The zebrafish model further provides an excellent system for testing multilocus variation genetic models [40] and future compound screenings in the search for precision medicine directed therapies for these severe disorders. Ethics All human research complied with all relevant ethical regulations and was approved by the relevant institutional review boards and the Ethical Committee of the University of Antwerp. Informed consents were obtained from all patients or their legal guardians in the respective centers where patients were recruited. Zebrafish experiments complied with all relevant ethical regulations and were approved by the Ethics Committee of the University of Leuven (Ethische Commissie van de KU Leuven, approval number ECD P150/2015) and by the Belgian Federal Department of Public Health, Food Safety and Environment (Federale Overheidsdienst Volksgezondheid, Veiligheid van de Voedselketen en Leefmileu, approval number LA1210199). Genetic and phenotypic analysis Molecular genetic analyses were performed in different research and diagnostic centers for which the details are given in Supplementary Notes. Families 3 and 6 were ascertained through the program GeneMatcher [24] . The seven novel VARS variants were all identified with WES or WGS in patients for whom standard diagnostic work-up failed to identify the cause of their neurodevelopmental phenotype. Variant filtering was done through locally developed pipelines taking into account the quality of the variant calling, presence in population databases, predicted impact on the encoded protein and segregation of the variants. VARS transcript NM_006295.2 was used for variant nomenclature. Clinical information was collected using standardized clinical templates that were completed by collaborating clinicians and geneticists. International League Against Epilepsy (ILAE) criteria were used for epilepsy syndrome classification when applicable [41] . In silico modeling of VARS variants The protein coding sequences of valyl-tRNA synthetases (VARS) were extracted from the UniProt server. The organisms and the UniProt accession numbers for their VARS sequences are as follows: Escherichia coli (E. coli), P07118; Thermis thermophilus (Thermis), P96142; Saccharomyces cerevisiae (yeast), P2637; Drosophila melanogaster (fruit fly), Q0E993; Caenorhabditis elegans (worm), Q23360; Danio rerio (zebrafish), F1Q740; Mus musculus (house mouse), Q9Z1Q9; Homo sapiens (human), P26640. Multispecies alignments were generated by use of Clustal Omega [42] . The alignment was further annotated in the protein ENDscript [43] with secondary structures derived from the structure of the ValRS-tRNA Val from Thermis thermophilus (PDB ID: 1IVS) as reported earlier [27] , [28] . The alignments were used to identify residues in the Thermis thermophilus complex corresponding to the residues altered by the VARS mutations, and then the resulting structures were rendered in space filling or stick representation using the program PyMOL (The PyMOL Molecular Graphics System, Version 1.2r3pre, Schrödinger, LLC). Isolation of patient-derived cell lines and cell culture Skin biopsies of patients 4 and 5 of family 3 (p.Leu78Argfs*35/p.Arg942Gln) and of a control individual were obtained following the local standard protocol and fibroblasts lines were generated. Fibroblasts, continuously kept at 37 °C in a humidified atmosphere with 5% CO 2, were cultivated in Dulbecco’s Modified Eagle Medium (DMEM), high glucose (Gibco) enriched with 10% heat-inactivated fetal bovine serum (Gibco), 1% l -glutamine (Life Technologies), 1% penicillin-streptomycin (Life Technologies). Lymphoblast lines were generated from fresh (peripheral) blood samples for patient 1, 2 and their parents (p.Leu434Val/p.Gly822Ser); and patient 9 (p.Arg404Trp) according to local standard protocol. The cells, continuously kept at 37 °C in a humidified atmosphere with 6% CO 2, were cultivated in RPMI 1640 Medium (Gibco), enriched with 10% heat-inactivated fetal bovine serum (Gibco), 1% l -glutamine, 1% penicillin-streptomycin and 1% sodium pyruvate (Life Technologies). Western blot Pelleted fibroblasts of patients 4, 5, and a control individual were homogenized in lysis buffer (20 mM Tris-HCl, pH 7.4, 2.5 mM MgCl 2 , 100 mM KCl, 0.5% NP-40) supplemented with protease inhibitors (Sigma), placed on ice for 30 min and cleared by centrifugation for 10 min at 20,800× g . Protein concentrations were determined using a Pierce BCA Protein Assay Kit (Thermo Fisher Scientific). Equal amounts of protein were diluted in NuPage LDS sample buffer 4X (Thermo Fisher Scientific) supplemented with 100 mM 1,4-dithiothreitol (DTT). Samples were denatured for 5 min at 95 °C. Subsequent size separation was performed with SDS-polyacrylamide gel electrophoresis on NuPAGE Novex 4–12% Bis-Tris gels (Thermo Fisher Scientific), which was later electrotransferred to a nitrocellulose membrane (GE Healthcare Lifescience). Membranes were blocked in 5% milk powder diluted in PBS-Tween 20 (0.1%) for 1 h. Primary antibody was incubated overnight at 4 °C or for 1 h at room temperature (RT) followed by secondary antibody for 1 h at RT. Visualization was effected with enhanced chemiluminescence detection using Amersham ECL Prime Western Blotting Detection Reagent (GE HealthCare) and an ImageQuantTM LAS4000 system (GE Healthcare Life Sciences). The density of the resulting bands, corrected for loading, was quantified using ImageJ and statistical significance assessed by one-way ANOVA with Bonferroni’s multiple comparisons test. The following primary antibodies were used: anti-VARS antibody (1:2500, Atlas Antibodies, HPA046710) and anti-alpha-tubulin (1:5000, Abcam, ab4074). The following secondary antibodies were used: anti-rabbit HRP-conjugated (1:10,000, Promega, W401B), anti-mouse HRP-conjugated (1:10,000, Southern Biotech, 1070–05). Uncropped scans of blots are available in Supplementary Figure 7 . qPCR of cycloheximide-treated cells Confluent T75 flasks of fibroblasts of patients 4, 5 and a control individual were treated for 6 h with (i) cycloheximide (CHX) (150 µg/mL), with (ii) dimethyl sulphoxide (DMSO) as a negative solvent control, or (iii) without treatment. After 6 h cells were collected, pelleted, and subsequently subjected to RNA extraction (Qiagen RNeasy Mini Kit), and followed by DNase treatment to remove residual genomic DNA (Turbo DNA free, Ambion). One microgram of total RNA was converted to cDNA using the Superscript® III First Strand Synthesis System (Life Technologies) with both oligo dT and random hexamer primers. Primers for real-time detection of VARS were custom-made (Supplementary Table 3 ) and a reaction mixture containing 20 ng cDNA template, primers and Power SYBR Green PCR Mastermix (Life Technologies) was amplified under cycling conditions according to the manufacturer’s protocol. Data were generated on a ViiATM7 Real-Time PCR system (Life Technologies) and analysed using Qbase + (Biogazelle) [44] . VARS transcripts were normalized against 4 housekeeping genes ( GAPDH, HPRT1, SDHA , and HMBS ). The ΔΔCq method was used to determine the relative levels of mRNA expression between experimental samples and controls. The results consist of data from at least two separate experiments where samples were run in triplicate. One-way ANOVA with Tukey’s multiple comparisons test was used to determine statistical significance. Immunocytochemistry For immunofluorescence (IF) staining of intracellular VARS protein, 50,000 fibroblasts of patients 4, 5 and a control individual were seeded on 12 mm diameter coverslips and 24 h later fixed with 4% paraformaldehyde (PFA) for 20 min at RT. Fibroblasts were permeabilized with 0.5% Triton X-100 in phosphate-buffered saline (PBS) for 2 min, blocked with 0.5% bovine serum albumin and 0.2% goat serum for 1 h and incubated overnight at 4 °C with following primary antibodies: anti-VARS protein (1:500; Atlas Antibodies, HPA046710), anti-KDEL (1:100; Enzo Life Sciences, 10C3), anti-Golgin-97 (1:200, Life Technologies, A21270), and anti-TOMM20 (1:200, Abcam, ab56783). With intermediate PBS washing steps, the secondary antibodies goat anti-rabbit IgG (Alexa Fluor 488) and goat anti-mouse IgG (Alexa Fluor 594) (both 1:500; Life Technologies) were added for 1 h at RT. Nuclei were stained for 10 min with Hoechst 33342 (1:10,000, Life Technologies). Coverslips were mounted (Dako) and images were taken with a Zeiss LSM700 confocal microscope using a ×63/1.40 plan-apochromatic objective. Possible cross-talk of the fluorescence channels was excluded by using frame-by-frame scanning. Aminoacylation assay Protein extracts containing aminoacyl-tRNA synthetase activity were prepared from ATTC control cells or patient-derived cell lines as described above. After washing twice with cold Dulbecco’s PBS, cells were lysed in 50 mM Tris-HCl, pH 7.5, 150 mM NaCl, 5 mM DTT, 0.5% Triton X-100, and protease inhibitor cocktail (Sigma). Protein concentration was measured by the standard Bradford assay. Aminoacylation assays were performed at 37 °C in 100 mM HEPES, pH 7.2, 30 mM KCl, 10 mM MgCl 2 with 107 μM total human placental tRNA, 2 mM ATP, 50 μM [ 14 C] valine (282.8 mCi/mmol), and were initiated by the addition of protein extract to a final concentration of 0.3 μg/µL of total protein. At three different time points over a 10-min interval, 5 µL aliquots were spotted onto 3MM Whatman filter papers presoaked with 5% TCA. The dried filters were washed three times with 5% TCA, once with 95% ethanol, then the radioactivity was quantitated by liquid scintillation. To calculate the specific activity of each sample, aminoacylation rates (pmol aminoacylated tRNA/min) were calculated from linear fits of the progress curve data, corrected for the total protein concentration. Yeast complementation assay VAS1 expression constructs for yeast complementation assays were generated using Gateway Cloning Technology (Invitrogen). The VAS1 gene (including the endogenous promoter sequence) was amplified from purified S. cerevisiae genomic DNA with primers bearing Gateway sequences. The resulting PCR product was BP-cloned into the pDONR221 entry vector per the manufacturer’s instructions. The BP reaction was used to transform E. coli , colonies were purified and subjected to Sanger sequencing to confirm sequence specificity and the absence of PCR-induced errors. Mutations assayed were generated using the QuickChange II XL Site-Directed Mutagenesis Kit (Stratagene) and variant-specific mutagenic primers (Supplementary Table 3 ). Mutagenesis reactions were performed on VAS1 pDONR221 constructs, which were subsequently transformed into E. coli . DNA from individual clones was purified and subjected to Sanger sequencing to confirm the presence of each mutation and to rule out PCR-induced errors. Two sequence-validated constructs each for wild-type VAS1 or the indicated mutations modeled in VAS1 (Fig. 2d ) were LR-cloned into pRS315 according to the manufacturer’s instructions. LR reactions were then used to transform E. coli , and colonies were purified and digested with BsrG1 (New England Biolabs) to confirm the presence of the respective VAS1 insert. Yeast complementation assays were carried out using a haploid S. cerevisiae strain with a deletion of the endogenous VAS1 locus. Viability of this strain was maintained via a pRS316 vector (including a URA3 gene) bearing a wild-type copy of VAS1 [45] . The haploid ∆ VAS1 strain was transformed with wild-type VAS1 , mutant VAS1 , or empty pRS315 bearing no VAS1 insert; pRS315 includes a LEU2 gene. Transformed yeast cells were selected for the presence of both vectors by growth on media lacking uracil and leucine. Two yeast colonies per transformation were selected for analysis and grown to saturation in 2 mL CM glucose broth (minus leucine and minus uracil) for 48 h at 30 °C. Cultures were either undiluted or diluted 1:10 or 1:100 in water. Subsequently, 10 μL of undiluted and diluted cultures were spotted on complete solid media containing 0.1% 5-fluoroorotic acid (5-FOA; Teknova) to select for spontaneous loss of the maintenance vector. Yeast viability was visually assessed after 3 days of incubation at 30 °C. Two colonies per transformation were assayed and each transformation was repeated three times using two independently generated constructs of either wild-type or the respective mutant VAS1 . Zebrafish husbandry All zebrafish ( Danio rerio ) lines used in this study were maintained at 28.5 °C on a 14 h light/10 h dark cycle under standard aquaculture conditions in a UV-sterilized rack recirculating system equipped with a mechanical and biological filtration unit. Fertilized eggs were collected via natural spawning and were raised in Danieau’s medium (1.5 mM HEPES, pH 7.2, 17.4 mM NaCl, 0.21 mM KCl, 0.12 mM MgSO 4 , 0.18 mM Ca(NO 3 ) 2 and 0.6 μM methylene blue) in an incubator on a 14 h light/10 h dark cycle at 28.5 °C. Whole-mount RNA in situ hybridization (WISH) One kb coding sequence fragment of vars was amplified from cDNA of AB wild-type strain (primers in Supplementary Table 3 ) and cloned into Zero Blunt® TOPO® PCR Cloning Kit (Invitrogen). Cloned DNA was linearized by XhoI and HindIII, then synthesized by SP6 RNA polymerase and T7 RNA polymerase using DIG RNA labeling kit (all Roche) for sense- and anti-sense DIG-labeled RNA probes, respectively. Embryos were fixed with 4% PFA, then washed with 1X PBS with Tween 20 (PBST), sequentially washed with 100–25% methanol and stored in 100% methanol at −20 °C until needed. On the first day of WISH, embryos were washed with 50–25% methanol, followed by 1X PBST. After treatment with proteinase K (Sigma) according to the developing stages, for permeabilization embryos were fixed again with 4% PFA and washed by 1X PBST. Embryos were hybridized in Hyb+ solution with the vars RNA probes at 70 °C overnight. On the second day, after serial washing with 2X SSCTw/50% formamide, 2X SSCT, 0.2X SSCT at 70 °C, embryos were blocked with 5% horse serum (Sigma) and incubated with anti-digoxigenin-AP Fab fragments (Roche) overnight at 4 °C. On the third day, embryos were developed with BCIP/NTP substrate (Roche). Staining was developed and stopped before the background signals started to appear in the embryos hybridized with the sense RNA probe. Generation of the vars CRISPR knockout zebrafish line A KO vars fish line was generated via CRISPR/ Cas9 technique [30] , [31] . vars sgRNA targeting exon 21 in the catalytic domain of vars protein (5′-CCGTCTCTAACAGTGTGCCC(GGG)-3′) was designed via GeneArt (Invitrogen) and further transcribed using MEGAshortscript™ T7 Transcription Kit (Ambion) and purified with MEGAclear™ Transcription Clean-Up Kit (Ambion). Cas9 (GeneArt CRISPR Nuclease mRNA) was purchased from Invitrogen. Single cell-stage fertilized wild-type embryos of AB line were injected with 7 pg vars sgRNA and 150 pg Cas9 mRNA (1 nL volume). The mutation at the target site was verified via Sanger sequencing. The remaining sgRNA/Cas9-injected embryos were raised till adulthood and outcrossed with WT adults. DNA extracted from F1 generation of 3 dpf whole larvae was screened for indels by Sanger sequencing. F0 founder with germline transmission and high rate of indels was selected to establish the knockout line. F1 generation embryos were raised to adulthood, fin clipped and sequenced. Individuals carrying the same mutation (4 bp deletion of GGGC) were identified and pooled together. All experiments were performed on embryos coming from F2 or F3 progeny. To confirm the genotype of the larvae, prior to or at the conclusion of an experiment, a whole larva or fin clip, respectively, was placed in separate tubes with 50 μL of lysis buffer (100 μM Tris, 10 μM EDTA, 0.7 mM proteinase K and 0.2% Triton X-100) to extract genomic DNA. Lysis was performed at 55 °C for 3 h, followed by 10 min at 95 °C. Lysed samples were genotyped by performing a PCR to amplify a 466 bp-region of interest (containing vars 4 bp deletion) using Titanium® Taq DNA Polymerase (Takara) and vars -specific primers (Supplementary Table 3 ). Successfully amplified PCR products were purified using ExoProStar (Illustra™) and Sanger sequenced with the same primers used for amplification. The genotypes of the individual larvae were analysed using SeqMan software (LaserGene). mRNA extraction and RT-qPCR for zebrafish studies Total RNA from 1, 3, and 5 dpf vars +/+, vars +/−, and vars−/− larvae, respectively, was extracted using TRIzol (Ambion, Life Technologies). Residual genomic DNA was removed by treatment with DNase I (Roche) with Protector RNase inhibitor (Roche). Reverse transcription of total RNA to single-stranded cDNA was performed on 1 μg of total RNA using the High Capacity cDNA Reverse Transcription Kit (Applied Biosystems) and further diluted 1:20. Real-time PCR was performed in HardShell ® Low-Profile Thin-Wall 96-Well Skirted PCR Plates (Bio-Rad) using CFX96 Touch Real-Time PCR Detection System (Bio-Rad). Primer and probe sequences for real-time detection of endogenous vars , as well as injected human WT VARS were custom-made (Supplementary Table 3 ). Reaction mixture containing diluted cDNA template, primers and 2x SsoAdvanced Universal SYBR Green Supermix (Bio-Rad) was amplified under cycling conditions according to the manufacturer’s protocol. Data generated were analysed using CFX Manager Software (Bio-Rad). vars transcripts were normalized against ribosomal protein S18 ( rps18) housekeeping genes that were experimentally determined to have the most stable expression in our reaction conditions. Primer and probe sequences for real-time detection of vars in Hi558Tg line were purchased from IDT (Supplementary Table 3 ). 2x TaqMan Universal Master Mix (ABI, USA) was used for the reaction. vars transcripts normalization was done against elongation factor 1-alpha ( ef-1 alpha ) and rps18 . The ΔΔCq method was used to determine the relative levels of mRNA expression between experimental samples and controls. The results consist of data from at least two separate experiments run in triplicate. One-way ANOVA with Tukey’s multiple comparisons test was used to determine statistical significance. Morphological studies in vars −/− zebrafish larvae Surviving vars +/+, vars +/−, and vars−/− larvae were counted daily and examined for major dysmorphologies, such as edema, head, and eye malformations, and for the presence of touch response, from 1 until 12 dpf. Dead larvae and all larvae from 12 dpf onwards were collected, stored at −80 °C and genotyped. For head size measurements, vars +/+, vars +/−, and vars−/− larvae were positioned in 3% methylcellulose. Lateral images of the head and the whole body of 3 and 5 dpf larvae were acquired using Leica MZ 10F fluorescence microscope with a Leica DFC310 FX digital camera and Leica Application Suite V3.6 software. Measurements were done blinded, manually in ImageJ software. Body length was measured from the anterior tip of the snout to the base of the posterior caudal fin. Head, brain, and eye areas were measured by tracing the boundary of the surface of interest using some predetermined spots on the head such as the otic vesicle or dorsal indentation just above the eye, at the level of the pineal gland. The absolute values of measured surface were normalized to the total body length of the larvae. Results were analysed using one-way ANOVA followed by Tukey’s multiple comparisons test. Histological analysis of vars −/− zebrafish larvae Fin clipped larvae were fixed in 4% PFA at 4 °C overnight and kept in 70% ethanol. At least five embryos or larvae per genotype group were embedded in 1% agarose in 1X TAE buffer. A mould, specifically designed to align zebrafish larvae, was used to produce agarose blocks with identical distributed wells of the same depth. Agarose blocks were gradually dehydrated in an enclosed automated tissue processor (Shandon Excelsior ES, Thermo Scientific) and subsequently embedded in paraffin. The heads of paraffin-embedded larvae were sectioned on a HM 325 manual rotary microtome (Thermo Fisher Scientific) at a thickness of 5 μm. The specimens were stained with hematoxylin and eosin (H&E stain) using Varistain™ Gemini ES Automated Slide Stainer (Thermo Fisher Scientific) according to laboratory protocols. The resulting sections were imaged at ×20 magnification in a SPOT 5.1 software (SPOT Imaging) by a SPOT-RT3 camera mounted on a Leica microscope. Brightness of the images was adjusted for the white background. Immunohistochemistry for active caspase-3 IHC detection of cell death was carried out on 5-μm-thick deparaffinised and rehydratated sections. Prior to IHC, the specimens were subjected to heat-induced antigen retrieval by incubation in 10 mM sodium citrate (pH 6.0) for 10 min at 98 °C, followed by a 30 min cool down and treatment with 3% hydrogen peroxide (2 × 8 min). The sections were blocked for 30 min in 5% normal goat serum in 1X TBST, and further incubated with primary antibody against active caspase-3 (BD Biosciences, Clone C92-605, 1:500 dilution) for 1 h at RT. After rinsing with 1X TBST, HRP-conjugated secondary antibody (Jackson ImmunoResearch, 111-035-003, 1:200 dilution) was applied for 1 h at RT. Next, the slides were treated with DAB+/chromogen (DAKO) for 1 min at RT and rinsed with deionized water. Nuclear counterstain was performed in hematoxylin for 3 min. After clearing in ethanol and histoclear, the slides were coverslipped under mounting medium. For each staining a negative control was included by processing sections in the absence of the primary antibody. The images were taken at ×40 magnification in a SPOT 5.1 software (SPOT Imaging) by a SPOT-RT3 camera mounted on a Leica microscope. Three to four equivalent sections were selected for each group and DAB positively stained nuclei were counted using Fiji. The results were expressed as percentage of apoptotic cells of the total cell number within a selected brain area. Results were analysed using one-way ANOVA followed by Tukey’s multiple comparisons test. Behavioral studies in vars −/− zebrafish larvae For the locomotor tracking, 3–7 dpf vars +/+, vars +/−, and vars−/− larvae were individually arrayed in a 96-well plate. After 30 min habituation, the larvae were placed in an automated tracking device (ZebraBox TM , Viewpoint, Lyon, France) and their locomotor behavior was followed for 1 h under dark conditions. The total movement was quantified using ZebraLab software (Viewpoint, Lyon, France) and expressed in actinteg units. The results were analysed by one-way ANOVA with Tukey’s multiple comparisons test. For the habituation assay, 6 dpf vars +/+, vars +/−, and vars−/− larvae were individually arrayed in a 96-well plate and equilibrated for 3 h in a uniformly illuminated testing chamber in an automated video-tracking device (ZebraBox TM , Viewpoint, Lyon, France). Further, they were exposed to a spaced training with light/dark cycles consisting of four blocks of 120 dark flashes (DFs) with 15 s interstimulus intervals (ISI) alternated with 10 min light periods. The increased movement during DFs was expressed in actinteg units. For the sake of clarity, standard deviations were not shown in the graph. Linear regression was used to find the best-fitting straight line through all the data points for each genotype group. Non-invasive local field potential recordings in vars −/− zebrafish larvae A larva was embedded in 2% low melting point agarose (Invitrogen). Recording electrodes were pulled from soda lime glass capillaries (1412227, Hilgenberg, Germany) on a DMZ Universal Puller (Zeitz, Germany) to a diameter of ~20 microns. It was filled with artificial cerebrospinal fluid (ACSF, 124 mM, NaCl, 2 mM KCl, 2 mM MgSO 4 , 2 mM CaCl 2 , 1.25 mM KH 2 PO 4 , 26 mM NaHCO 3 , and 10 mM glucose) and placed on larva’s head above the optic tectum. The recordings were performed using WinEDR (John Dempster, University of Strathclyde, UK). Differential signal was amplified 10,000 times by DAGAN 2400 amplifier (Minnesota, USA), band pass filtered at 0.3–300 Hz and digitized at 2 kHz via a PCI-6251 interface (National Instruments, UK). All the larvae used for LFPs displayed touch response. The duration of each recording was 10 min. An electrical discharge was classified as a positive event when its amplitude was at least three times the amplitude of the baseline, and had a duration of at least 100 ms. The analysis of the epileptiform events was done using automated detection software that was previously developed and validated by our group [46] . VARS rescue experiments Full-length wild-type human VARS cDNA (GenBank BC012808.2 from IRAUp969E0949D clone purchased from Source BioScience, UK) was cloned into a pCSDest vector (Addgene) using Gateway recombination technology according to the manufacturer’s instructions (Life Technologies) (WT VARS -pCSDest). Single nucleotide variants, leading to substitutions p.Gln400Pro, p.Arg942Gln, and p.Arg1058Gln at protein level, were introduced into WT VARS -pCSDest vector via site-directed mutagenesis using PWO SuperYield DNA polymerase (Roche) and primers containing given variants (Supplementary Table 3 ). Subsequent DpnI digestion was done to remove parental plasmid. All templates were verified by direct Sanger sequencing. Wild-type, p.Gln400Pro, p.Arg942Gln, and p.Arg1058Gln VARS mRNA was transcribed from linearized template plasmids using the SP6 mMessage mMachine® kit (Ambion) and purified by lithium chloride precipitation (Ambion). The rescue experiment was performed by cytoplasmic microinjection of 200 pg of WT or mutant VARS and GFP mRNA as control (1 nL volume) into 1-cell-stage vars−/− embryos. Following the injections, at 24 hpf only the healthy-looking embryos with normal morphology were selected for subsequent experiments (survival, behavioral tracking, and head measurements). Statistical analysis Data are presented as mean ± SD or mean ± SEM. Pairwise statistical significance was calculated with Student’s unpaired t -test or Mann–Whitney test for data that failed the normality test and multiple comparisons were determined with one-way ANOVA with Tukey’s test, using GraphPad Prism7 software.